Molecular mechanism of the wake-promoting agent TAK-925 The OX 2 orexin receptor (OX 2 R) is a highly expressed G protein-coupled receptor (GPCR) in the brain that regulates wakefulness and circadian rhythms in humans. Antagonism of OX 2 R is a proven therapeutic strategy for insomnia drugs, and agonism of OX 2 R is a potentially powerful approach for narcolepsy type 1, which is characterized by the death of orexinergic neurons. Until recently, agonism of OX 2 R had been considered ‘undruggable.’ We harness cryo-electron microscopy of OX 2 R-G protein complexes to determine how the first clinically tested OX 2 R agonist TAK-925 can activate OX 2 R in a highly selective manner. Two structures of TAK-925-bound OX 2 R with either a G q mimetic or G i reveal that TAK-925 binds at the same site occupied by antagonists, yet interacts with the transmembrane helices to trigger activating microswitches. Our structural and mutagenesis data show that TAK-925’s selectivity is mediated by subtle differences between OX 1 and OX 2 receptor subtypes at the orthosteric pocket. Finally, differences in the polarity of interactions at the G protein binding interfaces help to rationalize OX 2 R’s coupling selectivity for G q signaling. The mechanisms of TAK-925’s binding, activation, and selectivity presented herein will aid in understanding the efficacy of small molecule OX 2 R agonists for narcolepsy and other circadian disorders. Orexin signaling in the brain is the primary mechanism connecting diurnal circadian rhythms to arousal and wakefulness. Orexin A and B are neuropeptides (33 and 28 amino acids respectively, also known as hypocretins) derived from the preproorexin precursor and produced by a small set of dedicated neurons in the lateral hypothalamus, which stimulate release of neurotransmitters in diverse brain regions to promote wakefulness [1] . Orexin release is controlled by the circadian clock, and levels of orexin neuropeptides in mammalian cerebrospinal fluid follow a 24-hour cycle, peaking during the wake period [2] , [3] . The orexin peptides act by binding to the GPCRs OX1R and OX2R on target neurons to activate cellular signaling by G proteins and arrestins, particularly stimulating Gq/11-mediated release of calcium from the endoplasmic reticulum [4] . The human disorder narcolepsy type 1 is characterized by a deficiency of orexin signaling, resulting in a pentad of symptoms including excessive daytime sleepiness, disturbed nighttime sleep, hypnagogic/hypnopompic hallucinations, sleep paralysis, and cataplexy, a sudden loss of muscle tone triggered by strong emotions [5] . Narcolepsy type 1 affects approximately 100,000 adults in the U.S [6] ., and up to 3 million patients may be affected by the disorder worldwide. While the etiology of this disorder varies, the proximal cause of narcolepsy type 1 is the death of orexin neurons [7] . The resulting loss of orexin expression in the narcoleptic brain has been validated in human clinical studies [8] , and the causal relationship between orexin deficiency and the narcolepsy phenotype has been validated using preproorexin knockout mice and targeted killing of the orexin neurons [9] , [10] . Experiments in canine and mouse models also established that orexin control of circadian rhythms and wakefulness occurs predominantly through the actions of OX 2 R [11] , [12] , while signaling through OX 1 R is critical for stimulation of reward pathways [13] . These discoveries paved the way for small molecule drug discovery efforts targeting the orexin receptors in sleep/wake disorders, culminating in FDA approval of the dual orexin receptor antagonist (DORA) suvorexant (Belsomra®) for insomnia in 2014 [14] . Numerous small molecule chemotypes have been developed as DORAs or OX 2 R-selective antagonists [15] , however the discovery of small molecule OX 2 R agonists has lagged far behind, with very few potent lead compounds reported in the primary literature [16] or patents. A breakthrough in this area was recently achieved with the small molecule TAK-925 [17] , which displays low-nanomolar potency for OX 2 R activation and >5000-fold selectivity for OX 2 R over OX 1 R [18] . In animal studies, subcutaneous delivery of TAK-925 during the sleep period results in a dose-dependent increase in wakefulness and reduction in sleep time. TAK-925 is currently being explored as an orexin agonist in humans with narcolepsy, with multiple trials ongoing. Insights into the molecular basis for orexin receptor activation and inhibition have come from structural studies of OX 1 R and OX 2 R bound to different ligands. The first structure of OX 2 R with suvorexant revealed that the drug binds in a narrow membrane-embedded pocket analogous to the classic orthosteric site of adrenaline and beta-blocker binding in the β 2 -adrenergic receptor [19] . Structures of OX 1 R and OX 2 R with other antagonists showed that these compounds invariably bind to the same suvorexant site [20] , [21] , [22] . However, mutagenesis studies of the orexin receptors and other neuropeptide-activated GPCRs showed that interactions of the peptide agonists with the solvent-exposed extracellular loops (notably ECL2) are required to trigger full activation [23] , possibly underlying the difficulty in identifying small molecule agonist drug candidates. A recent cryo-EM study showed how a small molecule could mimic orexin B (OxB) to stabilize an active conformation of OX 2 R bound to a G protein [24] . In this work, we use cryo-EM of different OX 2 R-G protein complexes and associated pharmacological studies to understand the molecular mechanism of the drug candidate TAK-925. These structural and functional data reveal how TAK-925 activates OX 2 R with high potency and subtype selectivity, and with a preference for signaling through G q . Structure determination of TAK-925-bound OX 2 R coupled to G q and G i1 To capture active structures of OX2R bound to TAK-925, we purified complexes of the receptor together with heterotrimeric G proteins. Using recombinant protein from Sf9 insect cells, we elucidated the cryo-EM structure of OX 2 R coupled to a mini-G αs/q/iN /G β /G γ heterotrimer (referred to as OX 2 R-mG sqiN in this manuscript) in lauryl maltose neopentyl glycol (LMNG) micelles at 3.3 Å resolution (Supplementary Figs. 1a , b, and 2 ), serving as a model for the G q signaling complex leading to calcium release. In parallel, we solved the cryo-EM structure of OX 2 R coupled to a DNG αi1 /G β /G γ heterotrimer (referred to as OX 2 R-G i1 ) in digitonin at 3.2 Å resolution (Supplementary Figs. 1c , d, and 3 ), representing a G i signaling complex. Both cryo-EM efforts took advantage of scFv16 binding [25] , requiring generation of a modified mini-G s/q 71 [26] construct capable of binding the antibody fragment. The global cryo-EM envelope, atomic model, and density for TAK-925 in OX 2 R-mG sqiN are shown in Fig. 1a–c , while the analogous data for OX 2 R-G i1 are in Fig. 1d–f . Differences between OX 2 R models in these two structures are greatest at the G protein interface, although the models of the agonist-bound receptor are generally in close agreement, with a root mean square deviation (rmsd) of 0.7 Å. Both cryo-EM maps have well-defined sidechain density in the transmembrane region (Supplementary Fig. 4 ), and allowed placement and refinement of TAK-925 (Fig. 1c, f ). The stability of the modeled ligand conformation, particular regarding the saturated rings, was validated by quantum chemistry calculations (Supplementary Fig. 5 ). Fig. 1: Overall structures of the OX 2 R-G protein complexes. a Cryo-EM reconstruction of the complex OX 2 R-mG sqiN . Receptor density is in purple, TAK-925 is yellow, G αsqiN is orange, G β1 is green, G γ2 is pink. The cryo-EM density from Relion was displayed in Chimera as colored surfaces (contour level 0.033, 5 sigma), where different colored zones corresponded to the different polypeptides. b Model of complex as a cartoon, with the TAK-925 agonist as spheres with yellow carbons, blue nitrogens and red oxygens. c Cryo-EM density surrounding the ligand TAK-925 in the complex structure OX 2 R-mG sqiN , with the TAK-925 agonist as sticks with colored by heteroatom (yellow carbons, blue nitrogens and red oxygens). Cryo-EM density was displayed in Pymol (4.2 sigma) within 2 Å around TAK-925. d Cryo-EM reconstruction of the complex OX 2 R-G i1 . Receptor density is in purple, TAK-925 is yellow, G αi1 is blue, G β1 is green, G γ2 is pink. The cryo-EM density from cryoSPARC was displayed in Chimera as colored surfaces (contour level 0.5, 5 sigma), where different colored zones corresponded to the different polypeptides. e Model of complex as a cartoon, with the TAK-925 agonist as spheres with yellow carbons, blue nitrogens and red oxygens. f Cryo-EM density surrounding the ligand TAK-925 in the complex structure OX 2 R-G i1 , with the TAK-925 agonist as sticks with colored by heteroatom (yellow carbons, blue nitrogens and red oxygens). Cryo-EM density was displayed in Pymol (5 sigma) within 2 Å around TAK-925. Full size image Binding of TAK-925 to OX 2 R The molecular interactions between TAK-925 and OX 2 R are highly similar in the mG sqiN and G i1 complexes (Fig. 2a ), which solidifies the interpretation of the details of these interfaces. The cryo-EM density for the ligand binding pockets in the OX 2 R-mG sqiN and OX 2 R-G i1 complexes are shown in Supplementary Fig. 6a and b , respectively. TAK-925 adopts a compact, U-shaped conformation, contacting OX 2 R residues on TM2, TM3, TM5, TM6 and TM7 and burying 460 Å 2 of solvent-accessible surface area. The methyl carbamate and sulfonamide ‘arms’ of TAK-925 extend toward polar residues on either side of the orthosteric pocket, the latter group engaging in a hydrogen bond with Gln134 3.32 , while the phenyl-cyclohexane ‘tail’ projects deeper into the transmembrane region contacting Val138 3.36 , Phe227 5.42 , and Ile320 6.51 . TAK-925 and suvorexant share an overlapping binding site in OX 2 R despite having opposing ligand efficacy (Fig. 2b ). The diarylsulfonamide agonist Compound 1, reported in a previous cryo-EM structure [24] , shares elements of the TAK-925 pocket, but also extends further toward the extracellular loops of the receptor. Modulation of the position of Gln134 3.32 was previously observed in the OX 2 R-Compound 1 and OX 2 R-OxB complexes, and we similarly find that Gln134 3.32 undergoes the largest conformational switch of the orthosteric pocket residues with TAK-925 bound, compared to the suvorexant-bound inactive state (Fig. 2c ). Despite their very different chemotypes, TAK-925 and Compound 1 both have sulfonamides at similar positions in the active OX 2 R complexes (Fig. 2b ), which interact with Gln134 3.32 and promote a shifted position of TM3 (Fig. 2c ). The overall structure of active OX 2 R with TAK-925 is similar to active OX 2 R with Compound 1, with an rmsd of 0.6 Å, despite the use of a stabilizing extracellular nanobody in the Compound 1 complex. Fig. 2: Binding of TAK-925 to OX 2 R. a Overlay of contact residues (sticks with purple carbons for mG sqiN -coupled OX 2 R and sticks with blue carbons for G i1 -coupled OX 2 R) within 4 Å of TAK-925 (yellow carbons) when superimposing OX 2 R- mG sqiN and OX 2 R-G i1 . The OX 2 R backbone (silver) is from OX 2 R-mG sqiN . The hydrogen bond from Gln134 3.32 to TAK-925’s sulfonamide is not shown because this residue is behind the ligand from this viewpoint (same as in Fig. 2c ). b Overlay of TAK-925 (sticks with yellow carbons), Compound 1 (sticks with orange carbons) and suvorexant (sticks with cyan carbons) when superimposing the OX 2 R polypeptides from the OX 2 R-mG sqiN complex (this work), the OX 2 R-mini-G sqi complex ( PDB 7L1V ) and the antagonist-bound inactive conformation ( PDB 4S0V ). c Overlay of contact residues within 4 Å of TAK-925 when superimposing OX 2 R-mG sqiN (this work, magenta), OX 2 R-mini-G sqi /Compound 1 ( PDB 7L1V , orange) and the suvorexant-bound inactive conformation of OX 2 R ( PDB 4S0V , cyan). TAK-925 is shown as transparent spheres. d Stimulation of G q by OX 2 R wild type (WT) and mutants when bound to TAK-925 (top) and orexin B (bottom). Each data point represents an average from n ≥ 3 independent experiments (each performed in duplicate), where n is shown in Supplementary Table 2 . 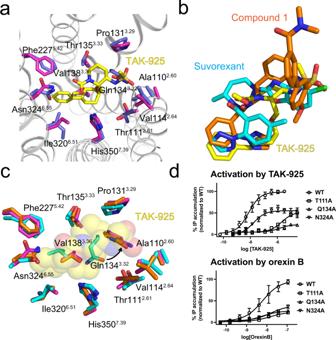Fig. 2: Binding of TAK-925 to OX2R. aOverlay of contact residues (sticks with purple carbons for mGsqiN-coupled OX2R and sticks with blue carbons for Gi1-coupled OX2R) within 4 Å of TAK-925 (yellow carbons) when superimposing OX2R- mGsqiNand OX2R-Gi1. The OX2R backbone (silver) is from OX2R-mGsqiN. The hydrogen bond from Gln1343.32to TAK-925’s sulfonamide is not shown because this residue is behind the ligand from this viewpoint (same as in Fig.2c).bOverlay of TAK-925 (sticks with yellow carbons), Compound 1 (sticks with orange carbons) and suvorexant (sticks with cyan carbons) when superimposing the OX2R polypeptides from the OX2R-mGsqiNcomplex (this work), the OX2R-mini-Gsqicomplex (PDB 7L1V) and the antagonist-bound inactive conformation (PDB 4S0V).cOverlay of contact residues within 4 Å of TAK-925 when superimposing OX2R-mGsqiN(this work, magenta), OX2R-mini-Gsqi/Compound 1 (PDB 7L1V, orange) and the suvorexant-bound inactive conformation of OX2R (PDB 4S0V, cyan). TAK-925 is shown as transparent spheres.dStimulation of Gqby OX2R wild type (WT) and mutants when bound to TAK-925 (top) and orexin B (bottom). Each data point represents an average fromn≥ 3 independent experiments (each performed in duplicate), where n is shown in Supplementary Table2. Error bars are ±SD. Data were normalized to the WT Emaxand fitted to the three-parameter model ‘log(agonist) vs response’ in GraphPad Prism 9. Source data are provided as a Source Data file. Error bars are ±SD. Data were normalized to the WT E max and fitted to the three-parameter model ‘log(agonist) vs response’ in GraphPad Prism 9. Source data are provided as a Source Data file. Full size image To further establish that the conformational switch seen for Gln134 3.32 is important for receptor activation, we carried out mutagenesis and measured G q signaling in an inositol phosphate (IP) accumulation assay (Fig. 2d , Supplementary Table 2 ). Consistent with the present and previous [24] structures, OX 2 R Q134 3.32 A loses almost all responsiveness to TAK-925 and OxB. In contrast, the N324 6.55 A mutant receptor can be activated by TAK-925, with an EC 50 (18 nM) close to the wild-type receptor (7.5 nM) in this assay (Fig. 2d , top panel), although this mutant has a lower E max likely due to lower plasma membrane expression (Supplementary Fig. 7 ). In the structure of OX 2 R-G i1 , N324 6.55 hydrogen-bonds to TAK-925’s carbonyl group with a distance of 2.7 Å between heteroatoms, however in OX 2 R-mG sqiN this distance is 3.3 Å. The non-ideal hydrogen bond between the ligand and OX 2 R helps explain why this contact is largely dispensable for TAK-925 signaling through G q (Fig. 3a ). Unlike TAK-925, OxB fails to activate the N324 6.55 A mutant (Fig. 2d , bottom panel), and the OX 2 R-OxB-G q complex [24] previously showed that the neuropeptide residue Thr27 makes a specific hydrogen bond to Asn324 6.55 . This polar residue was also previously demonstrated to be essential for antagonist binding and inhibition of OX 2 R in structural [19] , [20] and mutagenesis [27] studies. The residue Thr111 2.61 interacts with the ligand in the OX 2 R-mG sqiN structure such that the sidechain oxygen is 3.8 Å from TAK-925’s sulfonamide nitrogen. While the structure does not indicate a hydrogen bond between these groups, we found that mutation of this residue to alanine led to significantly reduced potency of the agonist (Fig. 2d , top panel, EC 50 2.1 μM). This loss of activity could be due to solvent-mediated effects, as discussed below. Finally, we carried out β-arrestin recruitment assays for a panel of OX 2 R mutants, and found that the residues important for TAK-925 activation of this pathway agree with the interactions that TAK-925 makes with the active OX 2 R orthosteric pocket in the cryo-EM structures (Supplementary Fig. 8 , Supplementary Tables 3 and 4 ). Notably, large reductions in β-arrestin recruitment by TAK-925 were measured for residues Gln134 3.32 as well as Tyr317 6.48 at the base of the orthosteric pocket, both of which undergo changes from the inactive to active conformations. Fig. 3: Structural basis for high selectivity of TAK-925 for OX 2 R. a Overlay of contact residues (sticks with purple carbons for mG sqiN -coupled OX 2 R and sticks with wheat carbons for inactive OX 1 R) within 4 Å of TAK-925 (transparent spheres with yellow carbons) when superimposing OX 2 R-G q and the antagonist-bound inactive conformation of OX 1 R ( PDB 4ZJ8 ). Divergent residues are circled by red dotted lines. b Stimulation of G q by OX 1 R wild type (WT) and subtype-swap single and double mutants when bound to TAK-925. Each data point represents an average from n = 3 independent experiments (each performed in duplicate). Error bars are ±SD. OX 1 R data were normalized to S103T/A127T E max . Data were fitted to the three-parameter model ‘log(agonist) vs response’ in GraphPad Prism 9. Source data are provided as a Source Data file. c Stimulation of G q by OX 2 R wild type (WT) and subtype-swap single and double mutants. Each data point represents an average from n ≥ 3 independent experiments (each performed in duplicate), where n is shown in Supplementary Table 2 . Error bars are ±SD. OX 2 R data were normalized to OX 2 R WT E max . Data were fitted to the three-parameter model ‘log(agonist) vs response’ in GraphPad Prism 9. Source data are provided as a Source Data file. Full size image From ligand structure-activity relationship (SAR) studies [17] , we found that critical determinants of TAK-925’s potency include the stereochemistry of substituents on the cyclohexane and piperidine rings, which enforces TAK-925’s stable U-shaped conformation seen in our structures (Fig. 1c, f , Supplementary Fig. 5 ). Furthermore, the sulfonamide of the ligand is essential for potency, and this group forms a tight polar interaction with the important residue Gln134 3.32 in the active state (Fig. 2a, c ). The SAR around the phenyl ring is narrow and replacement with aliphatic groups results in a reduction in potency, which is consistent with the phenyl-cyclohexyl tail of TAK-925 projecting into the deep hydrophobic pocket lined by nonpolar residues from TMs 3, 5, and 6. Selectivity of TAK-925 for OX 2 R over OX 1 R We have previously shown that TAK-925 has >5000 fold selectivity for OX 2 R over OX 1 R in calcium mobilization assays [18] . Our complex structures with TAK-925 show that, as with the DORA suvorexant [19] , [20] , the agonist contact sphere is highly conserved in OX 1 R, with only two substitutions: Thr111 2.61 →Ser and Thr135 3.33 →Ala (Fig. 3a ). It is possible that selectivity is enforced locally by these small differences in the respective binding pockets, however selectivity could also be the result of longer-range allosteric differences. To distinguish these possibilities, we carried out subtype swap experiments similar to what we previously performed for OX 1 R- and OX 2 R-selective antagonists [20] . When we mutated the two divergent binding pocket residues in OX 1 R to the corresponding amino acid in OX 2 R and carried out IP accumulation assays, we observed saturable activation by TAK-925 (EC 50 = 300 nM versus >100 μM non-saturating for wild-type OX 1 R). The two single mutants showed a partial increase (left-ward shift) in potency, indicating that both positions contribute towards selectivity (Fig. 3b ). Conversely, mutation of these two positions in OX 2 R to the corresponding amino acids in OX 1 R leads to a reduction (right-ward shift) in potency, and the double mutant results in EC 50 3.6 μM versus 7.5 nM for wild-type OX 2 R (Fig. 4c ). We also found that when OX 2 R Thr111 2.61 is mutated to alanine (instead of serine), receptor activation by TAK-925 is diminished (Fig. 2d top panel, EC 50 2.1 μM). Collectively, these data indicate that the high selectivity of TAK-925 for OX 2 R is largely caused by differences in the deep orthosteric pockets of the two receptor subtypes, rather than in the more divergent extracellular loops. If the active OX 1 R adopted a different conformation at the deep orthosteric pocket where TAK-925 binds, it would not be possible to rescue signaling with the S103T/A127T double mutant. Likewise, this result indicates that the allosteric pathway of activation for OX 1 R can be turned on by agonist binding at this site, and rules out the possibility that TAK-925 has minimal potency at OX 1 R due to differences in the allosteric transmission mechanism. Fig. 4: Propagated changes in OX 2 R activation. a Conformational changes of the side chains of key residues at the orthosteric site when bound to agonist, comparing the active conformation (purple sticks, transparent gray cartoon) and the inactive conformation (cyan sticks and transparent cyan cartoon). TAK-925 is shown as yellow sticks and suvorexant is in cyan sticks. b Overlay of PIF transmission switch in the active conformation of OX 2 R (purple sticks and transparent spheres) and the inactive conformation of OX 2 R ( PDB 4S0V , cyan sticks and transparent spheres). c Rewiring of micro switches on the intracellular side of OX 2 R when bound to agonist, comparing the active conformation (purple sticks, gray cartoon) and the inactive conformation (cyan sticks). TAK-925 is shown as yellow sticks. d Conformational changes of DRY motif when coupled to G protein, comparing the active conformation (gray cartoon and purple stick) and the inactive conformation (cyan sticks). The H5 helices of G q and G i are shown as orange and blue cartoon, respectively. Hydrogen bonds are shown as dotted lines. Full size image TAK-925 activation of OX 2 R How does TAK-925 stabilize the active conformation of OX 2 R? Compared to the inactive state, binding of TAK-925 causes a rotation in TM3 at the orthosteric pocket with sidechains moving towards TM2, including the shift of Gln134 3.32 described above. The ‘pull’ on TM3 occurs together with an opposing downward ‘push’ on Tyr317 6.48 induced by the deeper projection (relative to suvorexant) of TAK-925’s phenyl-cyclohexyl tail against TMs 3 and 6 (Fig. 4a ). This conformational change is disfavored by suvorexant due to the position of its benzoxazole, which packs against TM3 and prevents its rotation. A downward shift in the aromatic residue at position 6.48 (Ballesteros–Weinstein numbering [28] ) is observed in several active GPCRs, and has been suggested to initialize the hallmark outward rotation of TM6 during GPCR activation [29] . The signal is then further propagated down the receptor, where the ‘PIF switch’ (PVF in OX 2 R) [30] adopts an active conformation (Fig. 4b ), and the vacancy left by TM6’s outward movement is filled by the inward movement of TM7 toward TM3. In particular, the microswitch residue Tyr364 7.53 moves ~4 Å inward (Fig. 4c ) and sits between residues Leu145 3.43 , Ile148 3.46 , and Arg152 3.50 , while another microswitch residue Leu306 6.37 moves ~5 Å outward as a result of the repositioning of Arg152 3.50 . In parallel with the TM3-TM6-TM7 repacking, the ionic interaction between Asp151 3.49 and Arg152 3.50 is broken, and the cytosolic side of the receptor opens to accommodate the G protein α5 helix (Fig. 4d ). These latter conformational changes are also seen in other GPCRs [31] . OX 2 R-G protein interaction A major signaling cascade activated by the orexin neuropeptides in neurons is G q -mediated calcium release [32] . We were able to characterize TAK-925-bound samples of active OX 2 R with both mG sqiN (a G q mimetic) and G i1 , and are thus able to compare the interfaces between these complexes. The cryo-EM density for the receptor-G protein interface in the OX 2 R-mG sqiN and OX 2 R-G i1 complexes are shown in Supplementary Fig. 6c and d , respectively. A majority of the contacts occur between OX 2 R and the C-terminal α5 helix of each G protein (Fig. 5a, b ), as seen in previous activated receptor complexes [25] , [33] . The OX 2 R-mG sqiN interface has features similar to previously characterized GPCR-G q/11 complexes [34] , [35] , [36] , [37] . In particular, the end of the C-terminal α5 helix forms a ‘hook’ that packs against the TM7-Helix8 junction, and the sidechain of Tyr235 H5.23 from this hook extends across the center of the interface to form a hydrogen bond with ICL2 of the receptor (Ser164 ICL2 in OX 2 R, Figs. 4 d and 5a ). A similar interaction has been observed in other GPCR-G q complexes [36] , [37] , and Tyr235 H5.23 is not conserved in G i . Fig. 5: Interfaces of OX 2 R-G protein complexes and activation of G i and G q . a Interactions within 4 Å between OX 2 R and mG sqiN (gray cartoon and purple sticks for OX 2 R and orange cartoon and sticks for H5 helix of G q α subunit). Hydrogen bonds are dotted lines. b Interactions within 4 Å between OX 2 R and G i1 (gray cartoon and purple sticks for OX 2 R and blue cartoon and sticks for H5 helix of G i α subunit). Hydrogen bonds are dotted lines. c G q signaling mediated by OX 2 R with TAK-925 or orexin B. Each data point represents an average from n ≥ 3 independent experiments (each performed in duplicate), where n is shown in Supplementary Table 2 . Error bars are ±SD. Data were normalized to the orexin B E max and fitted to the three-parameter model ‘log(agonist) vs response’ in GraphPad Prism 9. Source data are provided as a Source Data file. d G i signaling mediated by OX 2 R with TAK-925 or orexin B. Each data point represents an average from 3 independent experiments (each performed in duplicate). Error bars are ±SD. Source data are provided as a Source Data file. Full size image The overall conformation of the OX 2 R-G i1 interface is similar to that of OX 2 R-mG sqiN (rmsd for receptor and Gα subunits together equals 1.3 Å). However, the OX 2 R-mG sqiN interface features more extensive contacts between OX 2 R and the mG αsqiN , resulting in burial of more surface area (1039 Å 2 versus 814 Å 2 ), Notably, the interaction of OX 2 R with the G i1 α5 helix is predominantly mediated by hydrophobic contacts, and G i1 makes only two polar contacts to the receptor’s polypeptide backbone (Fig. 5b ). In contrast, active OX 2 R makes 7 specific polar interactions with the mG αsqiN α5 helix, including from Ser164 ICL2 to Tyr253 H5.23 and from Thr302 6.33 to the mG αsqiN C-terminus (Fig. 5a , Supplementary Figs. 9 and 10 ). The backbone amide of Phe371 8.50 also hydrogen-bonds to Asn244 H5.24 of mG αsqiN (common G α numbering system [38] ) (Fig. 5a ), and this OX 2 R residue undergoes a downward shift during activation concomitant with the upward movement of Tyr364 7.53 (Fig. 4c ). To confirm whether OX 2 R can signal effectively through both G protein complexes, we carried out G q and G i signaling assays in HEK293 cells transfected with OX 2 R and G proteins. Both orexin B and TAK-925 showed poor ability to stimulate G i1 as measured by reduction in cAMP levels after forskolin treatment (Fig. 5d ). In contrast, both orexin B and TAK-925 induced robust G q -mediated IP accumulation with EC 50 values consistent with previous studies (8.2 nM and 8.1 nM, respectively) (Fig. 5c ). These results show that TAK-925 is similar to OxB in selectively activating G q signaling in cells. TAK-925 can fully activate OX 2 R despite its low molecular weight and non-peptidic structure. Earlier mutagenesis studies showed that residues on the ECL2 β-hairpin of OX 2 R are important for activation by OxB [23] , and we previously found that an α-helix preceding TM1 is involved in orexin binding [20] , which helps to position the neuropeptide C-terminal region to interact with the membrane-embedded site including N324 6.55 . These findings made it difficult to imagine how a drug-like small molecule could recapitulate the interactions needed to activate OX 2 R. Our present structures of active OX 2 R with TAK-925, along with the recent structure with Compound 1 [24] , explain how a low-MW drug can activate the receptor (Fig. 5d ) without fully mimicking the orexin neuropeptide. Indeed, TAK-925 binds in the same deep membrane-embedded site as the inhibitor suvorexant (Fig. 2a, b ), but is able to engage in concerted interactions with the receptor that stabilize the active conformation (Figs. 2 c and 4a ). The deep burial of TAK-925 at the membrane-embedded site also facilitates high affinity and potency, which the orexin neuropeptides can only achieve through multivalent contacts analogous to Class B GPCR/peptide interactions [39] . The mechanism of TAK-925 activation of OX 2 R sets a precedent that small molecule drug-like full agonists are possible even for the most challenging peptide-activated GPCR targets. Subtype selectivity remains a major challenge in GPCR drug development, both for agonists and antagonists [40] , [41] . TAK-925 has a high degree of OX 2 R selectivity, and this profile may be important to avoid OX 1 R activation of brain reward pathways associated with addiction [13] , while maintaining desirable sleep/wake effects. A typical strategy for achieving GPCR ligand selectivity is to exploit subpockets of the orthosteric site that are not conserved between subtypes, or to focus on more highly divergent allosteric sites [42] . Our structures of TAK-925-bound active OX 2 R and functional data (Fig. 3 ) show that subtype selectivity can be achieved even when the binding pockets are extremely highly conserved (19 out of 21 residues within 5 Å of TAK-925 are identical, with only Thr→Ser and Thr→Ala substitutions). How then does TAK-925 bind so much weaker to OX 1 R? As with OX 2 R-selective antagonists such as EMPA [21] , the contact sphere surrounding the ligand does not have to be very different between subtypes. Instead, we propose that small cavities resulting from the two smaller amino acids in a potential OX 1 R/TAK-925 complex lead to subtly diminished steric complementarity and less favorable desolvation upon surface burial [43] , with a large effect on binding free energy. These cavities are filled in the OX 1 R S103 2.61 T/A127 3.33 T double swap mutant, allowing for activation of this receptor by TAK-925. Other selective small molecule OX 2 R agonists such as Compound 1 [24] and the structurally similar YNT-185 [16] may also rely on the subtle differences between orthosteric pockets that are important for TAK-925, however the structure of Compound 1-bound OX 2 R shows that this type of diarylsulfonamide also makes contacts with the more divergent extracellular loops. Intriguingly, a recent medicinal chemistry effort [44] succeeded in making a potent dual orexin receptor agonist by modifying YNT-185 on the biphenyl moiety that is predicted to interact with the extracellular loops (given the structural analogy with Compound 1). This finding implies that OX 2 R-selective arylsulfonamide agonists may derive selectivity from interactions that are far from the TAK-925 interface. Determining the importance of different contacts for selectivity of this other agonist chemotype will require additional functional studies of mutant receptors. In the case of the antagonist EMPA, a previous structural and computational study [22] found that binding of a trapped ordered water molecule in a cavity formed at A127 3.33 of the putative OX 1 R complex is a major determinant of OX 2 R selectivity for this ligand. A similar phenomenon may occur to make TAK-925’s interaction with OX 1 R unfavorable, and will require computational approaches to elucidate. Our recent demonstration [45] of converting a dual selective antagonist (suvorexant) into an OX 1 R-selective antagonist by filling in this cavity with an aliphatic group suggests that modifying TAK-925 may be a viable strategy for creating OX 1 R-selective agonists. Few GPCRs have been rigorously characterized for their ability to activate multiple G protein classes, such as β 2 -adrenergic receptor coupling to G s and G i [46] . Several studies of OX 2 R using cAMP sensors or other engineered reporter assays have indicated that OX 2 R can also stimulate G s and G i signaling, although with reduced orexin potency [47] , [48] . From these studies, one may ask whether OX 2 R has any preference for activating a particular signaling cascade in cells or in vivo. Our structural data indicates that OX 2 R distinguishes between G q and G i , both in the extent of interaction and in the number of specific polar contacts (Fig. 5a, b , Supplementary Figs. 9 and 10 ). Meanwhile, our functional data shows that OX 2 R cannot substantially activate G i in HEK293 cells (Fig. 5d ), however the caveat remains that we did not measure this activity in transfected neurons. These results bolster observations that orexins function mainly by stimulating calcium release through activating G q [32] , [49] , and suggest that G protein promiscuity plays a limited role in orexin signaling. Several examples have recently been described of activated GPCR structures in complex with multiple G proteins (or G protein mimetics), which can provide insights into G protein selectivity. In most cases, the G protein known to couple most efficiently with the receptor has a larger buried surface area at the interface relative to subordinate G protein transducers [37] , [50] , which holds true for OX 2 R in this study (see above). The multivalent interactions between the receptor and the G protein are divergent, and selectivity is largely dependent on the unique features of each GPCR. In the GCGR-G s complex, ICL2 of the receptor engages more closely with G s compared to G i , and this interaction was demonstrated to be important for preferred G s coupling [50] . On the other hand, the GCGR-G i complex features unique contacts between ICL1 and G β and between ICL3 and G iα [50] . In the CCK1R-G q complex, ICL3 interacts with G αq and was shown to be important for G q coupling potency [37] . We do not observe a similar ICL3-G protein interaction in either of our OX 2 R-G protein complexes (Fig. 5a, b ), and the tip of ICL3 is disordered in both structures, however the caveat remains that we have used a G q mimetic (mG sqiN ) rather than wild-type G q protein in our study. In another example of multiple CCK1R-G protein structures, a different conformation was observed for the G protein α5 helix between mG sqi and G s complexes, which may reflect the potential for structural differences or dynamics of this key divergent G protein epitope to confer selectivity [36] . In our two OX 2 R-G protein structures, we observe highly similar conformations of the α5 helix (including the C-terminal ‘hook’) for the mG sqi and G i1 complexes (Fig. 5a, b , rmsd of 1.3 Å as described above). On the other hand, we find that our OX 2 R-G i1 interface is dominated by hydrophobic contacts, and the OX 2 R-G sqiN interface is a mixture of polar and hydrophobic interactions (Fig. 5a, b , Supplementary Figs. 9 and 10 ). A similar differentiation of interface properties is seen in comparing the preferential GCGR-G s complex to the GCGR-G i complex [50] . Intriguingly, several of the hydrogen bonds between OX 2 R and the mG sqiN α5 helix are conserved in CCK1R-G q structures: [36] , [37] Y235 H5.23 -S164 ICL2 and N231 H5.19 -A155 3.53 from OX 2 R-mG sqiN are analogous to Y391 H5.23 -Q153 ICL2 and N387 H5.19 -A142 3.53 in CCK1R-G q . This similarity may represent a shared contributor to G q selectivity for multiple GPCRs. An optimal drug for narcolepsy type 1 patients would be an oral pill that substitutes for deficient orexin neuropeptides and restores normal circadian patterns of orexin signaling, reversing debilitating symptoms such as sleep attacks and cataplexy [5] , [8] . This goal presents a complex set of pharmacokinetics challenges, since the drug must be orally bioavailable, brain penetrant, and have clearance kinetics on the order of hours. TAK-925 is administered intravenously (ClinicalTrials.gov NCT04091438), and more recently other small molecules have been discovered with improved oral absorption (ClinicalTrials.gov NCT04096560). The structures of active OX 2 R bound to TAK-925 presented here will help in understanding the important interactions that must be maintained to potently and fully activate the receptor by small molecule agonists. Chemicals The IUPAC name for TAK-925 is: [methyl (2 R ,3 S )−3-[(methylsulfonyl)amino]−2-{[( cis −4-phenylcyclohexyl)oxy]methyl}piperidine-1-carboxylate]. TAK-925 was synthesized by Takeda Pharmaceutical Company Limited or according to U.S. patent US20170226137. Compound was characterized as follows: mp: 113 °C; [α]D = + 16.3 (c 0.1, chloroform); 1H NMR (600 MHz, DMSO-d6): δ 1.40–1.55 (5H, m), 1.56–1.73 (5H, m), 1.87 (1H, brd, J = 13.2 Hz), 1.96 (1H, brd, J = 13.6 Hz), 2.44–2.57 (1H, m), 2.83 (1H, brs), 2.95 (3H, s), 3.40 (1H, brs), 3.53–3.62 (5H, m), 3.73 (1H, brt, J = 9.7 Hz), 3.84 (1H, brs), 4.47 (1H, brs), 7.15 (1H, brt, J = 7.2 Hz), 7.18 (1H, brs), 7.19 (2H, brd, J = 8.1 Hz), 7.27 (2H, brt, J = 7.4 Hz); 13 C NMR (151 MHz, DMSO-d6, the minor rotamer’s signals are marked with an asterisk): δ24.05, 24.39*, 26.00, 26.17*, 27.60*, 27.79, 28.68, 30.15*, 37.54, 38.13*, 39.91, 42.99, 51.01, 52.07, 53.90*, 54.49, 61.48, 61.89*, 71.68, 125.68, 126.51, 128.14, 147.34, 155.27*, 156.08; ESI/APCI MS (m/z): [M + H] + calcd. for C21H33N2O5S, 424.6; found, 425.2; analysis (calcd., found for C21H32N2O5S): C (59.41, 59.45), H (7.60, 7.59), N (6.60, 6.55). The sample used for structural biology and pharmacology studies was assessed to be >96% pure by LC-MS. Cloning and expression of the human OX 2 R-mG sqiN complex The cloning, expression, purification, cryo-EM data collection, and structure determination for the two OX 2 R-G protein complexes described in this paper were carried out independently. For the OX 2 R-mG sqiN complex the receptor construct contained residues 1–406 of wild-type human OX 2 R (OX 2 R 1–406 ). The C-terminal residues 407-444 of OX 2 R were removed to confer slightly improved expression and purification for this complex. Compared to wild-type OX 2 R, OX 2 R 1–406 displayed similar potencies for activation by TAK-925 and OxB (Supplementary Fig. 11 , Supplementary Table 2 ). The resulting construct was cloned into a modified pFastBac (ThermoFisher) baculovirus expression vector with the HA signal sequence followed by a FLAG tag at the N-terminus. We were unable to isolate a stable complex between OX 2 R and full-length wild-type G αq using the co-expression and purification strategy described below. Instead, an engineered G αq construct called mG αsqiN was made by modifying the chimeric G α protein ‘mini-G s/q 71’ previously described [26] . Briefly, the linker GGSGGSGG was deleted and residues 1–27 at the N terminus was replaced by residues 1–30 of G αi1 . A second pFastBac baculovirus was made with this mini-G αqiN gene. An additional pFastBac-Dual baculovirus was made with human G β1 and human G λ2 genes. An 8xHis tag was placed at the N-terminus of G λ2 . OX 2 R 1–406 , mG αsqiN , G β1 , and His 8 -tagged G λ2 were co-expressed in Spodoptera frugiperda (Sf9) cells with the addition of all three baculoviruses (ratio of 1 OX 2 R 1–406 :1 mG αsqiN :1G β1 G λ2 ) to Sf9 cells at a density of 3 × 10 6 per ml, along with 1 μM TAK-925 added to the media during growth. After 48 h, cells were harvested and stored at −80 °C. Cloning and expression of the human OX 2 R-G i1 -scFv16 complex The coding sequence of wild type human OX 2 R (residues 2–444) was synthesized and sub-cloned into pFastbac with an N-terminal FLAG tag followed by a fragment of β 2 AR N-terminal 1-24aa before OX 2 R, and a C-terminal 2xMBP-His 8 tag after OX 2 R. A TEV cleavage site was inserted between OX 2 R and the MBP tag. The prolactin precursor sequence was used as a signal peptide to increase protein expression. A dominant-negative bovine G αi1 construct called DNG αi1 was generated by site-directed mutagenesis to incorporate mutations G203A [51] and A326S [52] to decrease the affinity of nucleotide binding and increase the stability of the G αβγ complex. All three G protein complex components, human G αi1 , human G β1 and human G γ2 , were cloned into pFastbac individually. For OX 2 R-G i1 , scFv16 was cloned into pFastbac with a GP67 signal peptide at the N-terminal and a TEV cleavage-His 8 tag at the C-terminus. Baculoviruses for OX 2 R, DNG αi1 , His 8 -tagged G β1 , G γ2 , and scFv16 were co-expressed in Sf9 cells. Cell cultures were grown to a density of 3.5 × 10 6 cells/mL and infected with all five baculoviruses at a ratio of 1:1:1:1:1. 48 h after infection, cells were harvested and stored at −80 °C for further use. Cloning, expression and purification of scFv16 For OX 2 R-mG sqiN , scFv16 was expressed and purified separately. A synthesized DNA fragment encoding scFv16 [25] was cloned into pFastBac, with a melittin signal sequence at the N-terminus and a 10xHis tag at the C-terminus. The resulting construct was expressed in Sf9 cells. scFv16 was purified as previously described [53] . In brief, secreted scFv16 in the cell culture media was separated from Sf9 cells by centrifugation, and 10 mM Tris buffer pH 8.0 was added to balance pH. Then 1 mM Ni 2 SO 4 and 5 mM CaCl 2 were added to quench chelating agents. The media containing scFv16 was loaded onto Ni-NTA affinity resin by gravity, and the column was washed with 20 column volumes of buffer consisting of 50 mM HEPES pH 7.4, 150 mM NaCl and 10 mM imidazole. Protein was eluted from Ni-NTA resin with 10 column volumes of buffer consisting of 50 mM HEPES, 150 mM NaCl and 250 mM imidazole. The eluate was concentrated and run on a Superdex 200 gel filtration column. The peak corresponding to monomeric scFv16 was collected, concentrated and frozen until further use. Purification of the human OX 2 R-mG sqiN -scFv16 complex Cell pellets from 6L culture of the expressed OX2R-G q complex were resuspended and lysed for 30 min at 4 °C in a hypotonic buffer consisting of 10 mM HEPES pH 7.4, 160 μg/ml benzamidine, 100 μg/ml leupeptin,1 mM MgCl 2 , 0.1 mM TCEP, Apyrase (0.5 mU/ml, NEB) and 1 μM TAK-925. Lysed cells were spun down and homogenized using a dounce tissue grinder (Wheaton) in buffer consisting of 50 mM HEPES pH 7.4, 150 mM NaCl, 160 μg/ml benzamidine, 100 μg/ml leupeptin, 1 mM MgCl 2 , 1% (w/v) lauryl maltose neopentyl glycol (LMNG, Anatrace), 0.1% Na Cholate, 0.1% cholesteryl hemi-succinate (CHS, Steraloids), 10% glycerol, 0.5 mM TCEP, Apyrase (15 mU/ml, NEB) and 10 μM TAK-925. Solubilization proceeded for 1 hr at 4 °C, followed by centrifugation at 100,000 × g for 30 min at 4 °C. The supernatant was incubated with M1 anti-Flag affinity beads (Sigma) in batch-binding mode overnight at 4 °C in the presence of 2 mM CaCl 2 . After binding, the M1 beads were spun down and washed with 10 column volumes of buffer consisting of 50 mM HEPES pH 7.4, 150 mM NaCl, 0.05% LMNG, 0.005% Na Cholate, 0.005% CHS, 5% glycerol, 1 mM MgCl 2 , 2 mM CaCl 2 , 0.5 mM TCEP and 10 μM TAK-925. The complex was eluted from M1 beads with buffer consisting of 50 mM HEPES pH 7.4, 150 mM NaCl, 0.05% LMNG, 0.005% Na Cholate, 0.005% CHS, 5% glycerol, 0.5 mM TCEP, 10 μM TAK-925, 200 μg/ml FLAG and 5 mM EDTA. The eluted OX 2 R-G q complex was mixed with scFv16 at a molar ratio 1:1.2 and incubated for 30 min on ice. Finally, the mixture was concentrated and applied onto Superose 6 Increase 10/300 size exclusion column (GE Healthcare). The total yield of the complex was ~3 mg and the peak corresponding to the OX 2 R-mG sqiN -scFv16 complex was collected, concentrated and used in the following cryo-EM experiments (Supplementary Fig. 1a ). Purification of the human OX2R-G i1 -scFv16 complex Cell pellets from 10L culture were thawed at room temperature and suspended in 20 mM HEPES pH 7.2, 50 mM NaCl, 5 mM MgCl 2 . Complex was formed on membranes with addition of 10 μM TAK-925 and Apyrase (25 mU/mL, NEB), and incubation for 1.5 h at room temperature. Cell membranes were collected by ultra-centrifugation at 100,000 × g for 35 min. The membranes were then re-suspended and solubilized in buffer containing 20 mM HEPES, pH 7.2, 100 mM NaCl, 10% glycerol, 0.5% (w/v) n-Dodecyl β-D-maltoside (DDM, Anatrace), 0.1% (w/v) cholesteryl hemisuccinate TRIS salt (CHS, Anatrace), 0.1%(w/v) digitonin (Sigma) for 3 h at 4 °C. The supernatant was isolated after centrifugation at 100,000 × g for 45 min and then incubated overnight at 4 °C with pre-equilibrated Flag G1 resin (Genscript). After batch binding, the resin with immobilized protein complex was manually loaded onto a gravity column and washed with 10 column volumes of 20 mM HEPES, pH 7.2, 100 mM NaCl, 0.1% digitonin (w/v), 10 μM TAK-925. Protein was treated with TEV protease and eluted with the same buffer supplemented with 200 μg/ml flag peptide. Elution was concentrated and loaded onto a Superdex 200 10/300 GL increase column (GE Healthcare) pre-equilibrated with buffer containing 20 mM HEPES, pH 7.2, 100 mM NaCl, 0.075% digitonin, and 10 μM TAK-925. The total yield of the complex was ~5 mg and the eluted fractions of monomeric complex were collected and concentrated for cryo-EM experiments (Supplementary Fig. 1b ). Note that a different detergent was used for this complex compared to OX 2 R-mG sqiN -scFv16 (digitonin versus LMNG) because these purifications were developed independently, and not due to any specific preference of each complex for a different detergent micelle. Cryo-EM data acquisition for the OX 2 R-mG sqiN -scFv16 complex Prior to freezing grids, the OX2R-mG sqiN -scFv16 complex was concentrated to 9.5 mg/ml. Cryo-EM grids were prepared by applying 3.5 μl of this sample to glow-discharged Quantifoil R1.2/1.3 300-mesh Au holey carbon grids (Quantifoil Micro Tools GmbH, Germany), blotted for 4.5 s under 100% humidity at 4 °C and plunge frozen in liquid ethane cooled by liquid nitrogen using a Mark IV Vitrobot. SerialEM software was used for automated data collection. Images were recorded on a Titan Krios microscope (FEI) operated at 300 kV with a K3 direct electron detector (Gatan) in super-resolution correlated-double sampling counting mode using a slit width of 20 eV on a GIF-Quantum energy filter (Supplementary Fig. 12a ). Images were recorded at a nominal magnification of ×81,000, corresponding to a pixel size of 1.08 Å, and a target defocus range from −1.6 to −2.6 μm. Each movie stack was dose-fractionated over 32 frames for a total of 9 s under a dose rate of 8 e − /pixel/sec, resulting in a total dose of ~ 64 e − / Å 2 . Cryo-EM data acquisition for the OX 2 R-G i1 -scFv complex For cryo-EM grid preparation, 3 μl purified OX 2 R-G i1 -scFv16 complex at a concentration of 8 mg/mL was applied to an EM grid (Quantifoil, 300 mesh Au R1.2/1.3, glow discharged for 30 sec using a Solarus II plasma cleaner (Gatan)) in a Vitrobot chamber (FEI Vitrobot Mark IV). Protein concentration was determined by absorbance at 280 nm using a Nanodrop 2000 Spectrophotometer (Thermo Fisher Scientific). The Vitrobot chamber was set to 95% humidity at 4 °C. The sample was blotted for 2 s before plunge-freezing into liquid ethane. Cryo-EM movie stacks were collected on a Titan Krios microscope operated at 300 kV under EFTEM mode (Supplementary Fig. 12b ). Nanoprobe with 1 μm illumination area was used. Data were recorded on a post-GIF Gatan K2 summit camera at a nominal magnification of 130,000, using counting mode. Bioquantum energy filter was operated in the zero-energy-loss mode with an energy slit width of 20 eV. Data collection were performed using Leginon with one exposure per hole. The dose rate was ~8.4 e − /Å 2 /sec. The total accumulative electron dose was ~50 e − /Å 2 fractioned over 40 subframes with a total exposure time of 6 s. The target defocus range was set to −1.3 to −1.9 μm. Image processing of the OX 2 R-mG sqiN -scFv complex Data was processed in Relion 3.0 [54] following the same general protocol as previously described [53] . Dose-fractioned images were gain normalized, 2×2 Fourier binned, motion corrected, dose-weighted, and summed using MotionCor2 [55] . Contrast transfer function parameters were estimated using GCTF [56] . Approximately one thousand particles were picked manually and subjected to 2D classification. Representative projections of the complex were selected as templates for automated particle picking from all images. 8,929,023 extracted particles were 4×4 binned and subjected to 2D classification. A total of 2,661,363 particles were finally selected for 3D classification using the initial model generated by Relion as a reference. After 3 rounds of 3D classification, the classes showing good secondary structure features were selected, combined and re-extracted at the original pixel size of 1.08 Å. After 3D refinement and postprocessing, the resulting 3D reconstitution from 155,322 particles yielded a map at 3.3 Å resolution using the gold-standard FSC criterion (cryo-EM data-processing flowchart is shown in External Data Fig. 2 ). Local resolution map was calculated using Relion 3.0. Image processing of the OX2R-G i1 -scFv complex A total of 8453 movie stacks were collected. Each movie stack was aligned and dose weighted by 1.04 Å per pixel using MotionCor2 [55] . CTF parameters were determined using CTFFIND4 [57] . A total of 2,735,296 particles were auto picked using template picker and extracted with a box size of 256×256 pixels in cryoSPARC [58] . All particles were subject to two rounds of reference-free 2D classification. The following 2D classifications, 3D classifications and refinements were all performed in cryoSPARC. 677,124 particles were selected after two rounds of 2D classification based on the presence of intact complex. This particle set was used to do Ab-Initio reconstruction in four classes, which were then used as 3D volume templates for heterogeneous refinement. 332,173 particles were used for final non-uniform refinement. The global resolution of the final reconstruction is 3.13 Å (cryo-EM data-processing flowchart is shown in External Data Fig. 3 ). Local resolution map was calculated using cryoSPARC. Surface coloring of the density map was performed using UCSF Chimera [59] . Model building and refinement of the OX2R-mG sqiN -scFv complex The active structure of μOR ( PDB: 6DDF ) as well as structures of mini-G αq ( PDB: 6WHA ), G β1λ2 and scFv16 ( PDB: 6VMS ) were used as initial models for model rebuilding and refinement. A polyalaline model was made from the μOR structure, and together with structures of mini-G αq , G β1λ2 , and scFv16, components were docked into the cryo-EM density map in Chimera. The resulting model was subjected to autobuilding in Buccaneer [60] , iterative building in Coot [61] and refinement in Phenix.real_space_refine [62] . Initial coordinates and refinement parameters for the ligand TAK-925 were prepared with DRG web server ( http://davapc1.bioch.dundee.ac.uk/cgi-bin/prodrg ). MolProbity was used to evaluate the final structures. 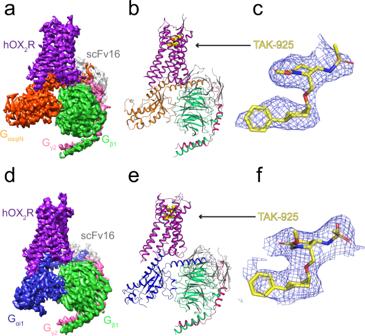In the Ramachandran plot, 97.6% and 2.4% of residues were in favored and allowed regions, respectively. Fig. 1: Overall structures of the OX2R-G protein complexes. aCryo-EM reconstruction of the complex OX2R-mGsqiN. Receptor density is in purple, TAK-925 is yellow, GαsqiNis orange, Gβ1is green, Gγ2is pink. The cryo-EM density from Relion was displayed in Chimera as colored surfaces (contour level 0.033, 5 sigma), where different colored zones corresponded to the different polypeptides.bModel of complex as a cartoon, with the TAK-925 agonist as spheres with yellow carbons, blue nitrogens and red oxygens.cCryo-EM density surrounding the ligand TAK-925 in the complex structure OX2R-mGsqiN, with the TAK-925 agonist as sticks with colored by heteroatom (yellow carbons, blue nitrogens and red oxygens). Cryo-EM density was displayed in Pymol (4.2 sigma) within 2 Å around TAK-925.dCryo-EM reconstruction of the complex OX2R-Gi1. Receptor density is in purple, TAK-925 is yellow, Gαi1is blue, Gβ1is green, Gγ2is pink. The cryo-EM density from cryoSPARC was displayed in Chimera as colored surfaces (contour level 0.5, 5 sigma), where different colored zones corresponded to the different polypeptides.eModel of complex as a cartoon, with the TAK-925 agonist as spheres with yellow carbons, blue nitrogens and red oxygens.fCryo-EM density surrounding the ligand TAK-925 in the complex structure OX2R-Gi1, with the TAK-925 agonist as sticks with colored by heteroatom (yellow carbons, blue nitrogens and red oxygens). Cryo-EM density was displayed in Pymol (5 sigma) within 2 Å around TAK-925. Statistics for data collection and refinement are included in Supplementary Table 1 . The cryo-EM density map has been deposited in the Electron Microscopy Data Bank under accession code EMD-25399 . Atomic coordinates have been deposited in the PDB under accession code 7SR8 . Structural figures were made using Pymol (Version 2.0 Schrödinger, LLC) and UCSF Chimera. Model building and refinement of the OX2R-G i1 complex The structures of OX 2 R ( PDB:5WQC ) and G i -scFv16 ( PDB: 6DDE ) were individually placed and rigid-body fitted into the cryo-EM map using Chimera. Manual inspection of the model was performed in Coot [61] , interspersed with restrained real-space refinement using Phenix.real_space_refine [62] . The ligand was placed by hand and then refined in Phenix. All regions of the model were checked thoroughly for registration correctness and fit to density during refinement. Statistics for data collection and refinement are included in Supplementary Table 1 . The cryo-EM density map has been deposited in the Electron Microscopy Data Bank under accession code EMD-25389 . Atomic coordinates have been deposited in the PDB under accession code 7SQO . Structural figures were made using Pymol and UCSF Chimera. Quantum chemistry calculation Northwest Computational Chemistry Package (NWChem) 6.8.1 [63] was used to perform all electronic structure calculations. All geometries were optimized at the B3LYP/6-31G* level of the Density-functional theory (DFT) in gas phase first and then with the solvation model based on density (SMD) model [64] in aqueous solution. Vibrational frequencies were computed in each case to confirm that each structure was a local minimum on the potential energy surface and to compute thermodynamic quantities. The standard Eckart projection algorithm, as implemented in NWChem, was applied to project out the translations and rotations of the nuclear hessian. Based on the frequencies obtained from the projected hessian, the zero point energy for the molecular system was calculated. Inositol phosphate accumulation assay for G q signaling The IP assay was adapted from a prior precedent [65] . HEK293 cells were maintained in DMEM-high glucose (Millipore Sigma) supplemented with 5% fetal bovine serum (Corning) and penicillin-streptomycin (Millipore Sigma). Receptor constructs used were the full-length wild-type (or mutant) human OX 1 R and OX 2 R sequences cloned into pCDNA3. To enhance the E max in the IP assay, a plasmid encoding full-length human G αq subunit [66] was co-transfected into HEK293 cells with plasmids encoding orexin receptor constructs using Lipofectamine 3000 (Thermo Fisher). 24 h after transfection, the cells were plated on poly-D-lysine coated (Millipore Sigma) tissue culture-treated 96 well white plates with clear bottoms (Perkin Elmer) at 30,000 cells per well in Inositol-free DMEM (MP Biomedicals) supplemented with 5% fetal bovine serum, 4 mM L-glutamine (Millipore Sigma), penicillin-streptomycin, and about 5 uCi (5 ul) per ml myo-[2-3H] inositol (Perkin Elmer). The following day, the media was replaced with agonists that were diluted in HBSS (Millipore Sigma) containing 10 mM lithium chloride (Millipore Sigma) and incubated at 37 °C for 45 min. Then agonists were removed and cells were lysed on ice for 30 min with 10 mM formic acid (Millipore Sigma). 1.25 mg of poly-lysine coated YSI SPA beads (Perkin Elmer) was added to each well. The plates were mixed on an orbital shaker for 30 min. The plates were read on a MicroBeta scintillation counter (Perkin Elmer) the following day. IP accumulation assays on different constructs were performed in n ≥ 3 independent experiments (each done in duplicate), where n is shown in Supplementary Table 2 . Cpm data were normalized to OX 2 R WT E max , and dose responses were fitted to the three-parameter model ‘log(agonist) vs response’ in GraphPad Prism 9 (GraphPad Software). Fitted pEC 50 values were analyzed for statistical significance compared to OX 2 R WT (with TAK-925 or orexin B) using one-way ANOVA followed by Dunnett’s test. All pharmacological parameters are displayed in Supplementary Table 2 . β-arrestin PathHunter assay β-Arrestin recruitment activity was measured by using the PathHunter system (DiscoveRX) according to the manufacturer’s instruction. Receptor constructs used were the full-length wild-type (or mutant) human OX 2 R sequences cloned into pCMV-ProLink (DiscoveRX). CHO-K1 cells stably expressing EA β-arrestin2 (DiscoveRX) were plated on 384 well white plates (Thermo Fisher) at 4000 cells/well in HamF12 (Wako Pure Chemical Industries) supplemented with 10% fetal bovine serum (Corning) and penicillin-streptomycin (Wako Pure Chemical Industries) and incubated overnight at 37 °C under 5% CO 2 . Cells were transfected with plasmids encoding wild type or each mutant ProLink-tagged human OX 2 R using FuGENE HD (Promega). The following day, the media was replaced with HBSS (GIBCO) containing 20 mM HEPES (GIBCO) and 0.1% BSA (Wako Pure Chemical Industries), and treated with TAK-925 for 2 h at 37 °C. Detection reagent was added and incubated for 1 h at room temperature. Luminescent signal was detected using an EnVision plate reader (PerkinElmer). β-arrestin assays on different constructs were performed in two or three independent experiments (each done in quadruplicate). Dose response curves (shown in Supplementary Fig. 8 ) were fitted to the three-parameter model ‘log(agonist) vs response’ in GraphPad Prism to determine pEC50 values. Fitted pEC 50 values were analyzed for statistical significance compared to OX 2 R WT (with TAK-925 or orexin B) using one-way ANOVA followed by Dunnett’s test. Inhibition of forskolin-stimulated cAMP production To measure G i signaling [67] , HEK293 cells were transfected with pGloSensor™−22F cAMP Plasmid (Promega) and CMV expression plasmid encoding human OX 2 R. To enhance the signal for the cAMP assay, we co-transfected a G i expression plasmid (CMV-driven) in which the full-length human G αi1 subunit sequence was cloned into pcDNA3. The following day, cells were harvested and washed with assay buffer, HBSS with 20 mM HEPES pH 7.4 (Millipore Sigma). Cells were suspended in assay buffer containing 0.5 mg/ml Luciferin (Gold Biotechnology) and plated on 96 well tissue culture-treated white plates with opaque bottoms (Thermo Fisher). The cells were incubated at 37 °C for 90 min. Forskolin (Millipore Sigma) diluted in assay buffer was added to wells for a final concentration of 5 mM. Luminescence was read at room temperature repeatedly in a CLARIOstar microplate reader (BMG Labtech) until the signal stopped increasing. Agonist diluted in assay buffer was added from a 7X stock and again the plates were read repeatedly until the signal was stable. Assays for either TAK-925 or orexin B were performed in 3 independent experiments (each done in duplicate). cAMP luminescence data were plotted as a fraction of the maximal signal with forskolin, and dose responses were fitted to the three-parameter model ‘log(inhibitor) vs response’ in GraphPad Prism 9 (GraphPad Software). Both TAK-925 nor orexin B (Fig. 5d ) displayed minimal diminution of cAMP signal comparable to cells without transfected OX 2 R. As a positive control, cells were transfected with pGloSensor™−22F cAMP, D2 dopamine receptor, and G αi1 plasmids, and tested for their response to dopamine (Millipore Sigma) after forskolin treatment. The measured IC 50 for dopamine was 4.9 ± 1.1 nM. Enzyme-linked immunosorbent assay (ELISA) for cell surface expression The cell surface expression levels of wild-type and mutant human OX 1 R and OX 2 R constructs were quantified by an enzyme-linked immunosorbent assay (ELISA). As above in IP accumulation and cAMP assays, wild-type and mutant human OX 1 R and OX 2 R constructs were cloned into pcDNA3. HEK293 cells were transfected with pCDNA3 expression plasmids encoding receptor constructs and full-length human G αq subunit, using Lipofectamine 3000 (Thermo Fisher). 24 h after transfection, the cells were plated on poly-D-lysine coated (Millipore Sigma) tissue culture-treated 24 well clear plates (Corning) at 200,000 cells per well in DMEM-high glucose (Millipore Sigma) supplemented with 5% fetal bovine serum (Corning) and penicillin-streptomycin (Millipore Sigma). After 24 h at 37 °C w/5% CO 2 , the media was aspirated and cells were washed with 200 μL/well of TBS buffer twice. 400 μL/well of 4% paraformaldehyde (PFA) were then added for fixation of cells, and cells were incubated for 30 min on ice. 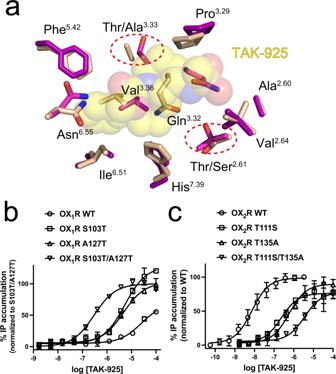Fig. 3: Structural basis for high selectivity of TAK-925 for OX2R. aOverlay of contact residues (sticks with purple carbons for mGsqiN-coupled OX2R and sticks with wheat carbons for inactive OX1R) within 4 Å of TAK-925 (transparent spheres with yellow carbons) when superimposing OX2R-Gqand the antagonist-bound inactive conformation of OX1R (PDB 4ZJ8). Divergent residues are circled by red dotted lines.bStimulation of Gqby OX1R wild type (WT) and subtype-swap single and double mutants when bound to TAK-925. Each data point represents an average fromn= 3 independent experiments (each performed in duplicate). Error bars are ±SD. OX1R data were normalized to S103T/A127T Emax. Data were fitted to the three-parameter model ‘log(agonist) vs response’ in GraphPad Prism 9. Source data are provided as a Source Data file.cStimulation of Gqby OX2R wild type (WT) and subtype-swap single and double mutants. Each data point represents an average fromn≥ 3 independent experiments (each performed in duplicate), wherenis shown in Supplementary Table2. Error bars are ±SD. OX2R data were normalized to OX2R WT Emax. Data were fitted to the three-parameter model ‘log(agonist) vs response’ in GraphPad Prism 9. Source data are provided as a Source Data file. Cells were washed with 200 μL/well of TBS buffer three times, followed by addition of 1% BSA. 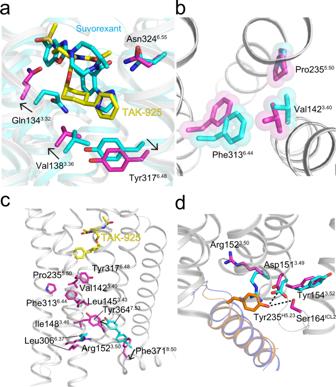Fig. 4: Propagated changes in OX2R activation. aConformational changes of the side chains of key residues at the orthosteric site when bound to agonist, comparing the active conformation (purple sticks, transparent gray cartoon) and the inactive conformation (cyan sticks and transparent cyan cartoon). TAK-925 is shown as yellow sticks and suvorexant is in cyan sticks.bOverlay of PIF transmission switch in the active conformation of OX2R (purple sticks and transparent spheres) and the inactive conformation of OX2R (PDB 4S0V, cyan sticks and transparent spheres).cRewiring of micro switches on the intracellular side of OX2R when bound to agonist, comparing the active conformation (purple sticks, gray cartoon) and the inactive conformation (cyan sticks). TAK-925 is shown as yellow sticks.dConformational changes of DRY motif when coupled to G protein, comparing the active conformation (gray cartoon and purple stick) and the inactive conformation (cyan sticks). The H5 helices of Gqand Giare shown as orange and blue cartoon, respectively. Hydrogen bonds are shown as dotted lines. 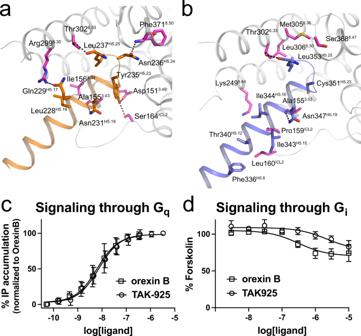Fig. 5: Interfaces of OX2R-G protein complexes and activation of Giand Gq. aInteractions within 4 Å between OX2R and mGsqiN(gray cartoon and purple sticks for OX2R and orange cartoon and sticks for H5 helix of Gqα subunit). Hydrogen bonds are dotted lines.bInteractions within 4 Å between OX2R and Gi1(gray cartoon and purple sticks for OX2R and blue cartoon and sticks for H5 helix of Giα subunit). Hydrogen bonds are dotted lines.cGqsignaling mediated by OX2R with TAK-925 or orexin B. Each data point represents an average fromn≥ 3 independent experiments (each performed in duplicate), wherenis shown in Supplementary Table2. Error bars are ±SD. Data were normalized to the orexin B Emaxand fitted to the three-parameter model ‘log(agonist) vs response’ in GraphPad Prism 9. Source data are provided as a Source Data file.dGisignaling mediated by OX2R with TAK-925 or orexin B. Each data point represents an average from 3 independent experiments (each performed in duplicate). Error bars are ±SD. Source data are provided as a Source Data file. Incubation proceeded for 1 h at room temperature. After 1% BSA in TBS was aspirated, 200 μL/well of 9.7 μg/ml of M1-Flag antibody (Sigma) in TBS w/1%BSA was added and cells were incubated at room temperature for 1 h. Cells were then washed with 200 μL/well of TBS w/1%BSA buffer three times, followed by addition of HRP-coupled secondary antibody with 1:2000 dilution in TBS w/1%BSA. Incubation proceeded for 1 h at room temperature. After cells were washed with 200 μL/well of TBS w/1%BSA buffer three times, 200 μL/well of TMB-ELISA (Thermo Fisher) was added. After a short time of incubation, 100 μL/well of colored solution was transferred to 96 well clear plates (Corning) containing 100 μL/well of 1 M H 2 SO 4 to stop reaction. Absorbance produced by HRP activity was immediately measured at 450 nm using a CLARIOstar microplate reader (BMG LABTECH). After measuring HRP activity, cells were washed with 200 μL/well of TBS twice and incubated with 200 μL/well of 0.2% (w/v) Janus green for 30 min. To remove extra Janus green, cells were washed with water three times, followed by addition of 800 μL/well of 0.5 M HCl. 200 μL/well of colored solution was transferred to the same 96 well clear plates (Corning). Absorbance at 595 nm was recorded by a CLARIOstar microplate reader (BMG LABTECH). For each well condition, the normalized cell surface expression was determined by dividing absorbance at 450 nm by absorbance at 595 nm. Experiments were repeated three times. The data were analyzed by one-way ANOVA (and Nonparametric or Mixed) and plotted as column with scattered points using GraphPad Prism 9 (GraphPad Software). Reporting summary Further information on research design is available in the Nature Research Reporting Summary linked to this article.